Sertoli cell-only phenotype and scRNA-seq define PRAMEF12 as a factor essential for spermatogenesis in mice Spermatogonial stem cells (SSCs) have the dual capacity to self-renew and differentiate into progenitor spermatogonia that develop into mature spermatozoa. Here, we document that preferentially expressed antigen of melanoma family member 12 (PRAMEF12) plays a key role in maintenance of the spermatogenic lineage. In male mice, genetic ablation of Pramef12 arrests spermatogenesis and results in sterility which can be rescued by transgenic expression of Pramef12 . Pramef12 deficiency globally decreases expression of spermatogenic-related genes, and single-cell transcriptional analysis of post-natal male germline cells identifies four spermatogonial states. In the absence of Pramef12 expression, there are fewer spermatogonial stem cells which exhibit lower expression of SSC maintenance-related genes and are defective in their ability to differentiate. The disruption of the first wave of spermatogenesis in juvenile mice results in agametic seminiferous tubules. These observations mimic a Sertoli cell-only syndrome in humans and may have translational implications for reproductive medicine. Mammalian spermatogenesis is a highly coordinated, dynamic process of cell differentiation with three distinc phases: mitois, meiosis, and spermiogenesis. Life-long testicular spermatogenesis depends on the presence of spermatogonial stem cells (SSCs) as well as their amplification and transition into progenitor and differentiating spermatogonia [1] , [2] . In mice, SSCs are derived from gonocytes that arise from primordial germ cells (PGCs) formed in the proximal epiblast during embryogenesis [3] , [4] , [5] , [6] . SSCs are located in the basal compartment of the seminiferous epithelium of the testis and have the capacity to divide which: (1) allows self-renewal to maintain the SSC pool; and (2) gives rise to progenitor spermatogonia, which have a large proliferative capacity, but are committed to differentiate [7] . SSCs reside in the population of A single (A s ) spermatogonia, which initiate mitotic divisions either to produce two new A s spermatogonia by complete cytokinesis or to generate chains of A paired (A pr ), and A aligned (A al(4) , A al(8) , A al(16) , and in rare cases, A al(32) ) spermatogonia (Fig. 1a ). Because of incomplete cytokinesis, A pr and A al cells are connected by intercellular bridges and represent undifferentiated spermatogonia [2] , [4] , [6] . The A al spermatogonia, as well as a few A pr spermatogonia, differentiate into A 1 spermatogonia without division and then mitotically divide five times to sequentially form A 2 , A 3 , A 4 , intermediate, and type B spermatogonia that are collectively termed differentiated spermatogonia [1] , [2] , [4] . Type B spermatogonia divide into two primary diploid spermatocytes, each of which meiotically divide into four haploid round spermatids to initiate spermiogenesis and form mature spermatozoa [2] . Fig. 1 Pramef12 is essential for spermatogenesis and male fertility. a The hierarchy of different cell types of spermatogonia during SSC self-renewal and differentiation. The A s spermatogonia are heterogeneous with SSCs and A s progenitors. The A s and A pr progenitors have the potential to become SSCs. A s spermatogonia produce chains of A pr A al(4) , A al(8) , and A al(16) undifferentiated spermatogonia that are connected by cytoplasmic bridges and are precursors of differentiated spermatogonia. b Fertility of > 3 pairs of Pramef12 Null and Pramef12 Het male and female mice mated 1:1. Mean litter sizes ± s.d. are shown with indicated genotypes. c Testes of P90 adult Pramef12 Null and Pramef12 Het mice. Scale bar, 1 mm. d Ratios of testis to body weight of Pramef12 Null and Pramef12 Het mice shown in c . Mean ± s.d, n = 6 biologically independent testes from six different animals. * P = 1.44E-08 by two-tailed Student’s t test. e Adult testis sections from Pramef12 Null and Pramef12 Het mice stained with periodic acid-Schiff (PAS) and hematoxylin. Pramef12 Null testes are agametic with a Sertoli cell-only phenotype. Scale bar, 50 μm. f Immunofluorescence of P90 adult testes from Pramef12 Null and Pramef12 Het mice after co-staining with antibodies to DDX4 (germ cells) and WT1 (Sertoli cells) as well as Hoechst 33342 (DNA). Scale bar, 50 μm. g Immunohistochemistry of P90 adult testes from Pramef12 Null and Pramef12 Het mice after staining with antibodies to cyclin D1 and PLZF. Arrowheads indicate positive-staining spermatogonia. Scale bar, 50 μm. h Quantification of cyclin D1-positive and PLZF-positive spermatogonia in Pramef12 Null and Pramef12 Het testes. Mean ± s.d, n = 3 biologically independent testes from three different animals. * P = 1.44E-28 (cyclin D1) and * P = 3.19E-26 (PLZF) by two-tailed Student’s t test. i Same as e , but of cauda epididymides. Representative of n = 6 c , n = 3 e , f , g , i independent biological replicates with similar results per condition Full size image A s SSCs represent 0.02–0.03% of all germ cells in the adult testes [8] . At present, three models for SSC renewal have been proposed [9] , [10] . In the classic A single model, the daughters of a dividing A s cell either contribute to maintenance of the SSC pool or begin to differentiate. In the fragmentation model, disintegration of larger clones (i.e., A aligned ) into single and pairs of cells significantly contribute to the maintenance of the SSC pool [11] , [12] , [13] , [14] , [15] . More recently, a hierarchical model proposes that restricted expression of ID4, PAX7, and/or BMI1 define a subset of spermatogonia as authentic stem cells [9] , [10] , [16] , [17] . Of note, few SSC marker proteins are specific to male germ cells and at present, mouse SSCs cannot be defined by the presence of a specific stem cell protein(s). FIGLA (factor in the germline, alpha) is a germline specific basic helix-loop-helix transcription factor required for mouse oocyte differentiation. Although expressed in male germ cells, Figla Null male mice appear normal and are fertile [18] . In a screen for downstream gene targets in the mouse ovary, PRAMEF12, a member of a PRAME multigene family, was identified [19] . Preferentially expressed antigen of melanoma (PRAME) was first discovered in human melanoma cell lines, and is a tumor-associated antigen recognized by cytolytic T lymphocytes [20] . The PRAME family genes, although present in humans and other mammals, are absent in zebrafish, amphibians, and invertebrates, indicating that the PRAME gene family is eutheria-specific [21] . The PRAME protein family belongs to a group of cancer-testis antigens that are aberrantly expressed in a variety of cancers and, in normal adult tissues, restricted to the testis and ovary [22] , [23] . Members of the PRAME gene family encode leucine-rich repeats, a structural motif frequently involved in protein–protein interactions [24] , [25] . It has been reported that PRAME family proteins function as transcription regulators in cancer cells and may play roles in spermatogenesis and oogenesis [26] , [27] . PRAME genes can be separated into groups according to their expression pattern in mice: testis ( Prame, Pramel1, Pramel 3 ) [26] , [28] , ovary ( Oogenesin1-4 ) [29] , [30] , [31] , embryo ( Pramel4-7 ) [32] , [33] , and both male and female gonads ( Pramel, Pramef8, Pramef12 ) [26] . However, the function of PRAME proteins remains unclear and no knockout mice have been reported. Using gene-edited mice, we now report the essential role of Pramef12 in maintaining SSC homeostasis and facilitating germ cell differentiation to ensure male fertility. Spermatogonial loss and infertility in Pramef12 Null mice To investigate the function of Pramef12 in germ cell development, we established PRAMEF12 null mice using CRISPR/Cas9. Two founder lines lacking either 37 or 49 bp after the start codon were obtained and bred to homozygosity (Supplementary Fig. 1a–d ). Pramef12 −/− female mice had normal fertility with litters the same size as Pramef12 +/− females when bred with Pramef12 +/− male mice. In contrast, Pramef12 −/− males were sterile and produced no pups when co-caged with either Pramef12 +/− or Pramef12 −/− female mice (Fig. 1b ). Pramef12 −/− males from each mutant line exhibited similar characteristics of testicular hypoplasia (Supplementary Fig. 1e, f ), and subsequent studies were focused on the line containing a 37 bp deletion, which we refer to as Pramef12 Null and use heterozygous null mice from the same line (designated Pramef12 Het ) as controls. Testes isolated from 3-month-old adult Pramef12 Null mice were significantly smaller and weighed less than controls (Fig. 1c, d ). Histologically, mutant seminiferous tubules were agametic and contained only somatic cells that resembled the Sertoli cell-only syndrome associated with human infertility (Fig. 1e ). The absence of germ cells was confirmed by immunofluorescence (IF) in which the germ cell-specific marker DEAD box polypeptide 4 (DDX4) was not detected, but Wilms tumor 1 (WT1), a Sertoli cell-specific marker, was observed (Fig. 1f ). Immunohistochemical analyses using antibodies for cyclin D1 (a marker for mitotically active spermatogonia) and promyelocytic leukemia zinc finger, PLZF (official name Zbtb16, a marker for undifferentiated spermatogonia) in control and Pramef12 Null testes indicate that cyclin D1-positive and PLZF-positive spermatogonia were rarely detected and their numbers were remarkably reduced in mutant testes (Fig. 1g, h ). No sperm were present in the cauda epididymides isolated from Pramef12 Null mice (Fig. 1i ) which, taken together, indicates that PRAMEF12 is essential for spermatogenesis. To determine the stage at which defects in spermatogenesis occurred, testes size and weight from control and mutant mice were compared from post-natal day 7 (P7) to P35 (Fig. 2a, b ). Histologic and immunohistochemical analyses with DDX4 staining document that mutant testes had normal numbers of spermatogonia at P2. However, spermatogonia were either completely depleted or significantly reduced in mutant seminiferous tubules by P7 (Fig. 2c–e ), revealing a defect in the proliferative expansion of spermatogonia that normally occurs during this period. To determine whether mutant spermatogonia could enter meiosis, P10 and P14 testicular sections were stained with PAS and P14 sections were stained with antibodies to γH2AX. Mutant testes contained γH2AX-positive spermatocytes although in diminished numbers, suggesting that mutant spermatogonia could enter meiosis (Fig. 2f, g ). From P14 to P35, testes from Pramef12 Null mice were significantly smaller in size and lower in weight than controls (Fig. 2a, b ). At P14, some mutant tubules were either devoid of germ cells or contained diminished numbers of spermatogenic cells (Fig. 2f, g ). These defects were more severe at P21, in which more than half of the Pramef12 Null tubules were agametic and the remaining tubules contained reduced numbers of germ cells (Fig. 2h ). At P35, when the first wave of spermatogenesis is complete, elongated spermatids and mature sperm were present in control testicular tubules and cauda epididymides. However, the mutant testes exhibited similar phenotypes as at P21 with few or no spermatogenic cells in seminiferous tubules, which contained numerous vacuoles (Fig. 2i, j ). No spermatozoa were present in mutant cauda epididymides despite of the presence of round and elongating spermatids in a few tubules (Fig. 2i, j ). Empty tubules depleted of germ cells were observed at P7, reached a maximum level at P21 and decreased at P35 in Pramef12 Null testes (Fig. 2k ). The spermatogenic cell loss was further confirmed by dual immunostaining with antibodies to DDX4 and WT1 in control and mutant developing testes from P14 to P35 (Supplementary Fig. 2a ). Terminal deoxynucleotidyl transferase dUTP nick end labeling (TUNEL) analysis exhibited a significant increase in apoptosis within mutant seminiferous tubules at P14 and P35 (Supplementary Fig. 2b, d ). However, the number of Sertoli cells in mutant testes did not differ from control testes (Supplementary Fig. 2a, c ). Fig. 2 Pramef12 is required for the first wave of spermatogenesis. a Morphology of testes from P14, P21, and P35 Pramef12 Null and Pramef12 Het mice. Scale bar, 1 mm. b Comparison of testes weight of P7, P14, P21, and P35 Pramef12 Null and Pramef12 Het mice. Mean ± s.d, n = 5 biologically independent testes from five different animals. * P = 3.81E-03 (P14), * P = 2.38E-06 (P21) and * P = 4.84E-08 (P35) by two-tailed Student’s t test. Immunohistochemistry c and immunofluorescence d staining of DDX4 in the testicular sections from P2 and P7 Pramef12 Null and Pramef12 Het mice. The merge in d is with Hoechst 33342 stained DNA. Scale bar, 50 μm. e Quantification of DDX4-positive cells per tubules in Pramef12 Null and Pramef12 Het testes at P2 and P7. Mean ± s.d, n = 3 biologically independent testes from three different animals. * P = 2.71E-07 by two-tailed Student’s t test. f Testicular sections of P10 and P14 Pramef12 Null and Pramef12 Het mice were stained with periodic acid-Schiff (PAS) and hematoxylin. Scale bar, 50 μm. g Immunofluorescence staining of γH2AX in testicular sections from P14 Pramef12 Null and Pramef12 Het mice. DNA was stained with Hoechst 33342. Arrows, pachytene spermatocytes (XY body); asterisks, Sertoli cell-only tubules. Scale bar, 50 μm. h , i PAS staining of P21 and P35 testes in Pramef12 Null and Pramef12 Het mice. The reduction in germ cell number becomes notable with the appearance of more agametic tubules (asterisks). Spermatogonia, 1; spermatocytes, 2; spermatids, 3; and elongated spermatozoa, 4; asterisks, agametic tubules. Scale bar, 50 μm. j Same as i , but of cauda epididymides. k Percentage of agametic tubules in Pramef12 Null testes from P7 to P35. Pramef12 Het control testes contain no empty tubules. Mean ± s.d, n = 3 biologically independent testes from 3 different animals at each age point. Representative of n = 5 a , n = 3 c , d , f – j independent biological replicates with similar results per condition Full size image To determine whether the sterility of P90 Pramef12 Null males arose from a lack of germline cells or a stage-specific block in spermatogenic differentiation, we extended our investigations of the Pramef12 Null phenotype from P48 to P75. Histological analyses documented that the defects in spermatogenesis were more severe in mutant testes which contained more agametic tubules and markedly diminished spermatogenesis from P48 to P75 compared with P35 Pramef12 Null testes (Fig. 2i , Fig. 3a–c ). Statistical analysis indicated that there was a significant age-dependent increase in the number of empty tubules from P35 to P90 (Fig. 2k , Fig. 3d ) that substantiates the conclusion that the sterility at P90 is owing to the absence of germ cells. Taken together, these observations indicate that Pramef12 deficiency causes a dramatic loss of spermatogonia and spermatogenic cells that disrupts the first wave of spermatogenesis in juvenile testes. This results in agametic seminiferous tubules in adult testes and male infertility. Fig. 3 Further evaluation of spermatogenic phenotype of Pramef12 Null mice. a Testicular sections of P48 Pramef12 Null and Pramef12 Het mice were stained with periodic acid-Schiff (PAS) and hematoxylin. Asterisks, agametic tubules. Scale bar, 50 μm. b Same as a , but of P60 testes. c Same as a , but of P75 testes. d Statistical analysis of empty tubules from P48 to P90 Pramef12 Null mice. Mean ± s.d, n = 3 biologically independent testes from three different animals at each age point. Representative of n = 3 a – c independent biological replicates with similar results per condition Full size image PRAMEF12 expression in spermatogonial cells RT-PCR documented that Pramef12 transcripts were largely restricted to the ovary and testis and were most abundant in P7 testes (Fig. 4a–c ). Using recently reported scRNA-seq data from adult mouse testis [34] , PRAMEF12 transcripts are not detected in adult Leydig, myoid, endothelial, macrophage cells, and barely detected in Sertoli cells. In contrast, PRAMEF12 is highly expressed in spermatogonia (~ 27-fold higher than in Sertoli cells) (Fig. 4d, e ). Moreover, PRAMEF12 transcripts are mainly expressed in spermatogonial subtype 1 (cluster 1), which corresponds to undifferentiated spermatogonia across the identified four spermatogonial subtypes in the adult mouse testis (Fig. 4f ). Our own scRNA-seq analysis of P7 mice confirmed these observations as will be described later in Results. Fig. 4 PRAMEF12 is specifically expressed in spermatogonia. a – c Abundance of Pramef12 transcripts in different adult tissues and P7 testes a , b and E17.5-P56 testes c was determined by RT-PCR a or qRT-PCR b , c using β-actin as a control. Molecular mass, left in a . The highest expression level of Pramef12 relative to β-actin was set to 1 in b , c . Mean ± s.d, n = 3 biologically independent samples per condition. d – f Analyses of the abundance of Pramef12 transcripts in 11 testicular cell types d , e and in cluster 1 of re-clustered germ cells f based on previously reported scRNA-seq data in adult mouse testes [34] . Numbers in d and the Y axis in e reflect the averaged UMIs detected in each individual cell. After re-clustering germ cells, Id4 , Plzf, and Sall4 serve as positive controls and, like Sall4 , Pramef12 was primarily enriched in the spermatogonial cluster 1, which corresponds to undifferentiated spermatogonia f . P value in f was obtained from the published scRNA-seq data [34] . Avg diff, log 2 -scale fold change. Percent of cells expressing gene in cluster 1 (Pct.1) or in non-cluster 1 cells (Pct.2). Exp and Exp + reflect mean expression of the marker in all cells of this cluster and in the marker-positive cells of this cluster, respectively. g Schematic representation of transgene expressing HA Pramef12 mCherry cDNA driven by the Pramef12 promoter (3.2 kb). h Whole-mount staining of P2, P7 and adult Pramef12 HA/mCherry testes with antibodies to mCherry (left), PLZF (middle) and merged (right). Scale bar, 50 μm. Examples of A s , A pr , and A al undifferentiated spermatogonia in adult testes (dotted circles) and enlarged (right panels). Arrowheads, high-light cytoplasmic location. Scale bar, 20 μm. i Same as h for P7 and adult testes, but with antibodies to mCherry (left), KIT (middle) and merged (right). Arrows, high-light co-localization of the two markers. j The expression profile of intracellular molecular markers for male germline cells. Except for NANOS2 (underlined), PRAMEF12 (underlined, red) is unique in its cell type specificity and is largely enriched in undifferentiated spermatogonia. Representative of n = 3 a , h , i independent biological replicates with similar results per condition Full size image To localize the protein in the absence of a commercially available antibody, we established Pramef12 HA/mCherry transgenic mouse line expressing Pramef12 cDNA tagged with HA and mCherry at the N- and C-termini, respectively (Fig. 4g ). Using a 3.2 kb Pramef12 promoter to drive expression of the recombinant protein and whole-mounts of P2, P7, and adult transgenic testes, cellular localization of PRAMEF12 was determined by confocal microscopy (Fig. 4h, i ). To define the identity and classification of PRAMEF12-positive cells, we co-stained PRAMEF12 with PLZF, which is a marker of undifferentiated spermatogonia, although it is also expressed in early stages of differentiation [35] . Immunostaining indicated that PRAMEF12 was expressed in the cytoplasm of spermatogonia and co-stained with PLZF in most undifferentiated spermatogonia at P2 and P7. Co-expression of PRAMEF12 and PLZF suggested that PRAMEF12 was possibly expressed in some A s , A pr , and chains of A al undifferentiated spermatogonia of adult Pramef12 HA/mCherry mouse testis (Fig. 4h ). A small fraction of undifferentiated spermatogonia were positive for PLZF without an mCherry signal (Fig. 4h ), indicating that the expression pattern of PRAMEF12 is consistent with molecular heterogeneity among undifferentiated spermatogonia [14] . To investigate expression of PRAMEF12 in spermatogonia poised to differentiate, we co-stained whole-mount testes with antibodies to KIT, a marker for differentiated spermatogonia. Co-expression of PRAMEF12 and KIT was detected in P7 seminiferous tubules (Fig. 4i ). PRAMEF12 and KIT also co-stained chained A al spermatogonia, but the abundance of PRAMEF12 was downregulated as spermatogonia further differentiated in adult Pramef12 HA/mCherry testis (Fig. 4i ). These observations suggest that PRAMEF12 persists and is co-expressed with KIT in clones of A al spermatogonia which are possibly in transition from undifferentiated to differentiating spermatogonia. In summary, PRAMEF12 is primarily enriched in undifferentiated spermatogonia, but is also present in some early KIT-positive differentiating spermatogonia in mouse testis (Fig. 4j ). PRAMEF12 is required for stem cell maintenance Because gonocytes re-enter mitosis shortly after birth, we determined the overall number of germ cells and undifferentiated spermatogonia from P2, P4, and P7 tubules after whole-mount staining with antibodies to DDX4 and PLZF. The number of DDX4-positive germ cells and PLZF-positive spermatogonia were comparable in control and Pramef12 Null tubules at P2. However, the number was substantially reduced in mutant tubules by P4 and P7 (Fig. 5a ), which was confirmed by morphometric analyses after staining with antibodies to PLZF (Supplementary Fig. 3a, d ). The number of GFRA1-positive spermatogonia was significantly decreased in mutant tubules as early as P4 at which time tubules without DDX4-positive germ cells were observed (Fig. 5b ). TUNEL assays indicated that the number of apoptotic spermatogonia in mutant testes was not significantly different from controls (Supplementary Fig. 3e, f ), suggesting that these defects were not primarily due to increased cell death. Fig. 5 Essential role of PRAMEF12 in early spermatogenic maintenance. a Immunofluorescence of whole-mount testes from P2, P4, and P7 Pramef12 Null (left group) and Pramef12 Het (right group) mice after staining with antibodies to DDX4 (left) or PLZF (middle) and merged (right). The number of PLZF-positive spermatogonia was comparable in P2 Pramef12 Null and Pramef12 Het tubules and significantly decreased in Pramef12 Null tubules as early as at P4, although still present at P7. Scale bar, 50 μm. b Same as a , but with antibodies to GFRA1 (co-receptor for GDNF) at P4. Asterisks, agametic tubules. c Same as a , but with antibodies to KI67 (marker of mitosis) and PLZF using whole-mount testes from Pramef12 Null (top) and Pramef12 Het (bottom) mice at P7. d The percent of KI67 + ; PLZF + double-positive among the total PLZF + single-positive spermatogonia in P7 Pramef12 Null and Pramef12 Het tubules. At least six random regions of individual testis were counted from at least three different mice. Mean ± s.d, n = 3 biologically independent samples per condition. * P = 5.89E-23 by two-tailed Student’s t test. Representative of n = 3 a – c independent biological replicates with similar results per condition Full size image Compared with controls, the average number of cyclin D1- and PCNA- (marker of proliferation) positive spermatogonia per tubule cross-section was significantly lower in mutant testes (Supplementary Fig. 3b–d ). Whole-mount co-staining for PLZF and KI67 (a marker for mitotic spermatogonia) in P7 seminiferous tubules also demonstrated that the number of PLZF + KI67 + spermatogonia was dramatically reduced in mutant tubules (Fig. 5c, d ). Immunoblots documented that expression of DDX4, PLZF, LIN28A (a marker for undifferentiated spermatogonia), and cyclin D1 was significantly decreased in P7 mutant testes compared with controls (Supplementary Fig. 3g ). Thus, the proliferative capacity of SSCs is impaired in Pramef12 Null mice, which leads to a defect in spermatogonial expansion that normally occurs in early post-natal testes. We also observed a significant and rapid reduction in the overall number of PLZF-positive and cyclin D1-positive spermatogonia in mutant testes from P14 to P35 mice (Supplementary Fig. 4a–d ). Overall, these results suggest that PRAMEF12 is required for SSC self-renewal and proliferation, and that disruption of Pramef12 impairs early spermatogenic maintenance and causes age-related decline of undifferentiated spermatogonial populations. PRAMEF12 is essential for spermatogonial differentiation To investigate the role of PRAMEF12 in spermatogonial differentiation, we determined that KIT-positive spermatogonia in both control and mutant seminiferous tubules were rarely detected at P2. However, the number of KIT-positive spermatogonia in mutant tubules was greatly diminished as early as P4 when a small portion of KIT-positive spermatogonia appeared in the control tubules. This expression pattern persisted and became more notable by P7 (Fig. 6a ). A marked reduction in the number of KIT-positive spermatogonia was also observed in sections of mutant testes at P7 (Fig. 6b ). These observations were confirmed by real-time RT-PCR and immunoblot, which documented that KIT mRNA and protein abundance was significantly reduced in P7 mutant testes (Fig. 6c, d ). Some mutant tubules exhibited spermatogonial arrest and failure of differentiation despite the presence of PLZF- and cyclin D1-positive spermatogonia at the basement membrane as evidenced by the absence of multiple stages of differentiating germ cells (Supplementary Fig. 4a, c ). These results suggest that although mutant testes contain a small population of PLZF- or cyclin D1-positive spermatogonia, these cells are unable to differentiate further. SOHLH1 and SOHLH2 have been implicated in coordinating spermatogonial differentiation [36] and the numbers of SOHLH1- and SOHLH2-positive spermatogonia were markedly decreased in mutant seminiferous tubules compared with controls by P7 (Fig. 6e ). Taken together, these data indicate that PRAMEF12 has an important role in spermatogonial differentiation. Fig. 6 Essential role of PRAMEF12 in spermatogonial differentiation. a Immunofluorescence of whole-mount testes from P2, P4, and P7 Pramef12 Null and Pramef12 Het mice after staining with antibodies to DDX4 (left) or KIT (middle) and merged (right). KIT-positive spermatogonia were rarely detected at P2 in either Pramef12 Null or Pramef12 Het tubules but were present at P4 and increased at P7 in Pramef12 Het tubules. Few KIT-positive spermatogonia (arrow) were observed in P7 Pramef12 Null tubules. Scale bar, 50 μm. b Immunohistochemistry of sections from P7 Pramef12 Null (top panels) and Pramef12 Het (bottom panels) testes after staining with antibodies to DDX4 (left) or KIT (middle) and merged with Hoechst 33342 to stain DNA (right). Arrowheads, KIT-positive cells in Pramef12 Null testes. Scale bar, 50 μm. c Quantitative real-time RT-PCR of Kit mRNA abundance in P7 Pramef12 Null and Pramef12 Het testes using β-actin as an internal load control and setting the abundance in Pramef12 Het testis to 1. Mean ± s.d, n = 3 biologically independent samples per condition. * P = 1.43E-05 by two-tailed Student’s t test. d Immunoblot of KIT protein in P7 Pramef12 Null and Pramef12 Het testes using α-tubulin as a load control. e Same as a , but with antibodies to SOHLH1, SOHLH2, and PLZF. The number of spermatogonia positive for SOHLH1 and SOHLH2 was significantly reduced in P7 Pramef12 Null tubules (top panels). Representative of n = 3 a , b , d , e independent biological replicates with similar results per condition Full size image Recombinant PRAMEF12 rescues Pramef12 Null male mice We sought to use the Pramef12 HA/mCherry transgenic mice to rescue the defects in spermatogenesis and fertility of Pramef12 Null mice. Pramef12 HA/mCherry transgenic mice crossed into Pramef12 Null mice had decreased testicular size and weight compared with either Pramef12 Het or Pramef12 Het ;Pramef12 HA/mCherry littermates, but were comparable to Pramef12 Null littermates (Supplementary Fig. 5a, b ). About 20% of the seminiferous tubules in Pramef12 Null ;Pramef12 HA/mCherry males contained spermatogenic cells and a few mature sperm were present in the cauda epididymis (Supplementary Fig. 5c, d ). Because of the low efficiency of rescue, we generated a second transgenic mouse line in which recombinant PRAMEF12 was tagged with FLAG-6xHis and HA at the N- and C-termini, respectively (Supplementary Fig. 5e ). Pramef12 Null ;Pramef12 FLAG/6xHis/HA rescue males had significantly larger testis size and weight compared with Pramef12 Null littermates, albeit slightly smaller than Pramef12 Het or Pramef12 Het ;Pramef12 FLAG/6xHis/HA mice (Supplementary Fig. 5f, g ). Restoration of all stages of spermatogenesis was observed in Pramef12 Null ;Pramef12 FLAG/6xHis/HA seminiferous tubules with normal numbers of mature sperm in the cauda epididymides (Supplementary Fig. 5h, i, k ). Although the abundance of Pramef12 and Eomes mRNA in the Pramef12 Null ;Pramef12 FLAG/6xHis/HA testis was only partially restored at P7 (Supplementary Fig. 5j ), Pramef12 Null ;Pramef12 FLAG/6xHis/HA males had normal fertility when mated with Pramef12 Null females (Supplementary Fig. 5k ). Overall, these data suggest that recombinant PRAMEF12 can substitute for the endogenous protein to rescue spermatogenesis and fertility in Pramef12 Null mice despite only partial restoration of the protein. Pramef12 deficiency affects spermatogenic gene expression To investigate the molecular consequences of the loss of Pramef12 , we compared the transcriptomes of Pramef12 Null and Pramef12 Het testes at P2 and P7. RNA-seq analysis identified 11 upregulated and 70 downregulated genes at P2 using adjusted P < 0.1 (Fig. 7a ). Gene ontology (GO) analysis documented that downregulated transcripts were significantly enriched for those that function in RNA metabolic processes, stem cell population maintenance (e.g., Sall1 , Ascl2 , Lin28a , Pou5f1 , Esrrb , Sall4 , Piwil2 ), reproductive process, spermatogenesis (e.g., Ddx4 , Adcy10 , Tdrd1 , Bnc1 , Stra8 ), gene silencing and cell differentiation (e.g., Cdh1 , Foxc2 , Stra8 , Sox3 ) (Fig. 7b ). Some known transcripts (e.g., Utf1 , Plzf , Gfra1 , Sall4 , Foxc2 , Sox3 ) involved in SSC maintenance and differentiation were significantly reduced in P2 mutant testes (Fig. 7c ). Using the same criterion, we found that 1599 genes were upregulated and 2147 genes were downregulated in P7 mutant testes (Fig. 7d ). Among downregulated genes at the two time points, most of the genes (68/70) downregulated at P2 were also significantly downregulated at P7 and Pramef12 Null testes at P7 showed a substantially higher number of downregulated genes (Fig. 7f ). The genes significantly downregulated at P7 included those involved in cell cycle (222 genes), regulation of gene expression (572 genes), RNA processing (159 genes), meiotic cell cycle (53 genes), reproductive process (239 genes), spermatogenesis (87 genes including Ddx4 , Adcy10 , Dazl , Taf7l , Tdrd1 , Rnf17 , Mael , Btbd18 ), stem cell population maintenance (31 genes including Ascl2 , Esrrb , Sall1 , Eomes , Utf1 , Pou5f1 , Lin28a , Sall4 , Gfra1 , Ret , Plzf ) as well as cell differentiation (263 genes including Dmrtb1 , Kit , Stra8 , Dnmt3b , Rarg , Sohlh1 , Sohlh2 ) (Fig. 7e, g ). We next verified the expression patterns of the genes by real-time RT-PCR at P7. The qRT-PCR results confirmed significant downregulation of two stemness-related genes ( Pou5f1 , Lin28a ), seven genes involved in SSC maintenance ( Pramef12 , Utf1 , Eomes , Sall4 , Gfra1 , Ret , Plzf ), seven genes involved in spermatogonial differentiation ( Dmrtb1 , Stra8 , Kit , Sohlh1 , Rarg , Dnmt3b , Sohlh2 ) and six genes involved in spermatogenesis ( Piwil2 , Piwil1 , Dazl , Ddx4 , Btbd18 , Tdrd1 ) (Fig. 7h ). Taken together, these data suggest that Pramef12 deficiency globally influences the expression of genes that control multiple spermatogenic processes, including SSC maintenance and differentiation. Fig. 7 Pramef12 deficiency alters expression patterns of spermatogenic genes. a MA plot (log ratio RNA abundance versus abundance) of RNA-seq data from Pramef12 Null and Pramef12 Het testes at P2. 11 genes and 70 genes were upregulated and downregulated, respectively, in Pramef12 Null testes using adjusted P < 0.1 as the cut off. b Gene ontology of downregulated genes in P2 Pramef12 Null testes. Genes that support stem cell population maintenance indicated in red text fly-out. GO terms were obtained by GOrilla analysis. P value was obtained from the data by GOrilla analysis. c Genes related to stem cell maintenance and differentiation that were significantly downregulated (log 2 -fold change) in P2 Pramef12 Null testes. d Same as a , but at P7. In all, 1599 genes and 2147 genes were upregulated and downregulated in Pramef12 Null testes, respectively. e Same as b , but at P7. P value was obtained from the data by GOrilla analysis. f Venn diagram depicting the overlap of downregulated genes determined at two developmental time points, P2 and P7. g RNA-seq results of selected transcripts (log 2 -fold change) related to SSC maintenance, differentiation and spermatogenesis that were significantly downregulated in P7 Pramef12 Null testes. h Quantitative RT-PCR validation of downregulated genes involved in SSC maintenance, differentiation and spermatogenesis in Pramef12 Null testes at P7. For comparison, the abundance (relative to β-actin ) of each gene in Pramef12 Het control mice was set to 1. Data are presented as mean ± s.d for n = 3 biologically independent samples per condition Full size image scRNA-seq defines the transcriptome of Pramef12 Null testes To address the cellular heterogeneity of spermatogonia, we isolated single cells from six testes of P7 Pramef12 Het and Pramef12 Null mice, respectively, and performed scRNA-seq analysis using the 10X Genomics platform (Fig. 8a ). From a total of 5473 Pramef12 Het and 5116 Pramef12 Null testicular cells, 5221 and 4839 cells passed standard quality control and were retained for subsequent analysis (Supplementary Fig. 6a ). On average, we detected 7446 unique molecular indices (UMIs) and 2450 genes in each individual cell, which are sufficient to define distinct cell types in mouse testis. Fig. 8 Single-cell transcriptome of Pramef12 Het and Pramef12 Null testicular cells. a Schematic illustration of the workflow for scRNA-seq analysis. b tSNE and clustering analysis of combined single-cell transcriptome data from P7 Pramef12 Het and Pramef12 Null testicular cells. Each dot represents a single-cell and cell clusters are distinguished by colors. c Dotplot for expression of selected marker genes across all identified cell types. d Gene expression patterns of selected somatic cell marker genes projected on the tSNE plots. e Expression patterns of marker genes for germ cells visualized in tSNE plots. Pramef12 is exclusively expressed in germ cell population but not in somatic cell populations Full size image Unsupervised clustering of the total 10,060 testicular cells projected onto t-distributed stochastic neighbor embedding (tSNE) analysis plots identified nine major cell types (Fig. 8b ). None of the clusters consisted of cells derived solely from either Pramef12 Het or Pramef12 Null testes (Supplementary Fig. 6b ). Cluster identity was assigned based on expression patterns of known marker genes in mouse testis (Fig. 8c–e , Supplementary Fig. 6c, d , Supplementary Data 1 ). We identified a germ cell population expressing spermatogonia-specific genes and eight somatic cell populations including five known somatic cell populations: Sertoli, myoid, Leydig, endothelial, and macrophages and three new cell populations: a cell cycle-related cell population and two unknown cell populations expressing fibroblast-specific marker genes including Col1a1 , Col3a1 , Pdgfra, and Dlk1 . Pramef12 was primarily expressed in the germ cell population and was not expressed in somatic cell populations (Fig. 8c, e ) consistent with previous findings in adult mouse testis [34] . Transcriptome signatures of Pramef12 Null testes To determine the transcriptome-wide signatures of SSC development and how PRAMEF12 effects this process, we re-clustered the 1153 Pramef12 Het and 654 Pramef12 Null spermatogonial cells. Uniform Manifold Approximation and Projection (UMAP) and marker gene analyses were performed for cell type identification [37] . Based on UMAP, we observed four distinct spermatogonial subtypes/states. Pseudotime analysis provided an arrow vector, which aligned with the developmental order of germline stem cells from spermatogonial state 1 to state 4 (SPG1 to SPG4) (Fig. 9a ). None of the clusters/states derived solely from Pramef12 Het or Pramef12 Null spermatogonial cells (Supplementary Fig. 7a ). Differentially expressed genes (DEGs) were observed among the four clusters and several classic spermatogonial marker genes for each state were identified in our single-cell data (Fig. 9b , Supplementary Fig. 7b , Supplementary Data 2 ). Gene ontology analysis identified the top several terms for these DEGs in each of the SPG1-4 states (Supplementary Fig. 7c ). Marker gene analysis suggests that SPG1 cells correspond to SSCs, as they highly express SSC marker genes including Id4 , Etv5 , Gfra1 , Lhx1, and Ret (Fig. 9b ). SPG2 cells express Ddit4 , Utf1 , Egr4 , Pramef12 , Sall4, and Plzf and display low expression of differentiation markers (Fig. 9b , Supplementary Fig. 7d ) consistent progenitor/undifferentiated spermatogonia. In contrast, SPG3 cells express high levels of early differentiation marker genes such as Kit , Stra8 and Dnmt3b and low levels of Pramef12 , Sall4 and Plzf (Fig. 9b , Supplementary Fig. 7d ) which indicates that this cell population is likely early differentiating spermatogonia. SPG4 cells mainly express late differentiation marker genes including Prss50 and Ly6k and high levels of early meiotic genes such as Hormad1 and Prdm9 (Fig. 9b ), implicating them as differentiated spermatogonia. Therefore, the expression patterns of spermatogonial marker genes recapitulate the developmental order of germline cells from SPG1 to SPG4. In addition, we found that the expression pattern of Pramef12 is similar to Sall4 , Plzf , Lin28a and Sdc4 in spermatogonia (Supplementary Fig. 7d ). Fig. 9 Transcriptome-wide signatures of germline stem cell development. a Focused analysis (UMAP clustering and pseudotime ordering) of combined (left), Pramef12 Het (middle), and Pramef12 Null (right) germ cells documented four biological subtypes following the order of SPG1 to SPG4 (state 1 to state 4). b Gene expression patterns of selected marker genes corresponding to each cellular state on the UMAP plots. c Summary schematic depicting the percentage of spermatogonia in each cellular state in Pramef12 Null and Pramef12 Het testes. Pramef12 deficiency significantly impairs germline stem cell development as determined by the decreased percentage of differentiated cells in SPG3 and SPG4. d Differentially expressed genes (DEGs) between Pramef12 Null and Pramef12 Het cells in SPG2, SPG3, and SPG4. Log 2 FC, log 2 -fold change. Null and Het indicate the percentage of cells in which the gene was detected in Pramef12 Null and Pramef12 Het samples, respectively. e UMAP plots of the expression patterns of selected DEGs in SPG2 subtype in Pramef12 Null and Pramef12 Het samples Full size image We determined that 22.2%, 11.0%, 44.7%, and 22.2% cells sorted into SPG1, SPG2, SPG3, and SPG4, respectively, in Pramef12 Het sample and 35.5%, 29.9%, 16.3%, and 18.3% cells sorted into SPG1, SPG2, SPG3, and SPG4, respectively, in Pramef12 Null sample (Fig. 9c ). A dramatic decrease in the percentage of SPG3 and SPG4 cells in the Pramef12 Null sample suggests that Pramef12 deficiency severely impairs germline stem cell development. Identification and analysis of differentially expressed genes between Pramef12 Null and Pramef12 Het cells in SPG subtypes revealed that Utf1 , Nanos3 , Sall4 , Gfra1, and Ret , required in maintaining the undifferentiated spermatogonial population, and Stra8 , important for spermatogonial differentiation, were significantly reduced in mutant SPG2 cells (Fig. 9d , Supplementary Data 3 ). Consistently, genes related to spermatogonial differentiation such as Stra8 and Dnmt3b , were markedly downregulated in mutant SPG3 cells. Although Prss50 , Stra8 , Syce3 , Syce2 , Tex101 , Rhox13, and Ly6k were largely decreased in mutant SPG4 cells (Fig. 9d , Supplementary Data 3 ). These results further demonstrate that Pramef12 -deficient spermatogonia exhibit lower expression of several SSC maintenance- and differentiation-related genes. Moreover, differential expression analysis of the expression patterns of above genes further documented that the percentage of cells expressing several SSC maintenance-related genes in SPG2 in Pramef12 Null cells was sharply reduced and cells expressing differentiation marker genes in SPG3 and SPG4 were significantly downregulated compared with Pramef12 Het cells (Fig. 9d, e , Supplementary Fig. 7e ). Taken together, single-cell transcriptional analysis of male germline cells indicates that PRAMEF12 is crucial for germline stem cell maintenance and differentiation. SSC fate in Pramef12 Null mice A recent study documents the developmental kinetics and transcriptome dynamics of SSC specification in the spermatogenic lineage [38] . To define the SSC fate in the absence of PRAMEF12, we combined the published scRNA-seq data on germ cells isolated from P0, P3, and P6 testes [38] with our scRNA-seq data on P7 Pramef12 Het and Pramef12 Null germ cells, and re-clustered the spermatogonial cells. We observed six distinct spermatogonial subtypes/states based on UMAP and differential gene expression (Fig. 10a ). The identity of each state was determined by the age distribution of cells in each cluster and spermatogonial marker genes (Fig. 10a–d ). P0 cells (86.6%) were mainly enriched in SPG1 and SPG2, which expressed high levels of SSC markers Id4 , Etv5 , Ret, and moderate levels of Lhx1 . P3 cells (64.9%) were primarily sorted into SPG3 and SPG4 that possessed high levels of SSC-associated markers including Id4 , Etv5 , Ret , and Lhx1 . 10.6% cells clustered into SPG1 and SPG2, and 24.6% cells clustered into SPG5 and SPG6 corresponding to differentiated spermatogonia. P6, P7 Pramef12 Het , and P7 Pramef12 Null cells shared some overlap among the clusters and were primarily represented by clusters 3-6. Cluster 5 possesed low levels of SSC-associated markers, high levels of progenitor markers ( Neurog3 , Sox3 ) and low levels of terminal differentiation markers ( Kit , Stra8 ), identifying them as progenitor spermatogonia formed from the SSC pool. Cluster 6 possesed the lowest levels of SSC-associated markers and the highest expression of terminal differentiation markers ( Kit , Stra8 ), which characterized them as more differentiated spermatogonia. Based on the above analyses of known markers, the developmental trajectory of SSCs is from SPG1 to SPG6. Interestingly, the distribution of cells in cluster 5 in P7 Pramef12 Null cells is much higher than in P0 (40.6% versus 1.4%), in P3 (40.6% versus 6.5%), in P6 (40.6% versus 25.8%), and in P7 Pramef12 Het (40.6% versus 26.0%) cells (Fig. 10d ), suggesting that a higher percentage of progenitor spermatogonia were present in Pramef12 Null testes. This indicates that in the absence of PRAMEF12, the SSCs had lower stem cell potential and more closely resembled progenitor spermatogonia, which is supported by the transcriptome analyses in which a higher percentage of cells remained as progenitor spermatogonia. This implies that Pramef12 deficiency significantly impairs stem cell potential and blocks stem cell differentiation at an early stage of spermatogenesis consistent with our findings (Fig. 9 ) that Pramef12 deficiency impedes germline stem cell development. Fig. 10 Spermatogonial stem cell fates in Pramef12 Null male mice. a UMAP clustering of the combined germ cells including P0, P3, P6, P7 Pramef12 Het , and Pramef12 Null samples documented six biological subtypes following a developmental trajectory of SPG1 to SPG6 (upper left). Five additional UMAP plots specific to each individual sample (right and below). b Gene expression patterns of selected spermatogonial marker genes corresponding to each cellular state on the UMAP plots: SPG1 ( Id4 , Etv5 , Ret ); SPG2 ( Id4 , Etv5 , Lhx1 , Ret ); SPG3 ( Id4 , Etv5 , Lhx1 , Ret ); SPG4 ( Id4 , Etv5 , Lhx1 , Ret ); SPG5 ( Neurog3 , Sox3 ); and SPG6 ( Kit , Stra8 ). c Dotplot representation of average scaled expression and the percentage of cells within each cluster for selected marker genes across all ages and cell types. d Table of the distribution and the percentage of the cells within each cluster and each sample Full size image Mammalian spermatogenesis is a dynamic process that is sustained by a balance between maintaining a population of self-renewing SSCs and the ability of these cells to differentiate into mature spermatozoa. Abnormalities in this equilibrium lead to spermatogenic failure and male infertility. Here, we introduce PRAMEF12 as an important regulator of spermatogonial biology that is expressed in undifferentiated and early differentiating spermatogonia. We document that genetic ablation of Pramef12 impairs SSC self-renewal and early differentiation, which prevents sustained cycles of spermatogenesis and results in a Sertoli cell-only syndrome in adult mice. Comparative bulk and scRNA-seq data provide evidence that Pramef12 deficiency dysregulates previously reported SSC maintenance- and differentiation-related genes and results in impaired germline stem cell development. Comparison with normal transcriptomes of SSCs further demonstrates that Pramef12 deficiency significantly impairs stem cell potential and blocks stem cell differentiation. Taken together, these data conclusively establish PRAMEF12 as an essential factor in maintenance of the spermatogenic lineage in the testis, which is essential to ensure robust spermatogenesis and male fertility. Previous studies have identified molecular markers at defined stages of undifferentiated stem and progenitor spermatogonia (Fig. 4j ). Except for NANOS2, all are expressed in other tissues and presumably have additional roles in development. Within the testes, expression of ID4, BMI1, PAX7, and EOMES is restricted to a subset of A s spermatogonia [39] , [40] , [41] . GFRA1, UTF1, and NANOS2 are limited to A s , A pr , and short A al spermatogonia [42] , [43] , [44] , whereas PLZF, SALL4, LIN28A, CDH1, and FOXO1 are expressed later in undifferentiated cells as well as in early differentiated spermatogonia [14] , [45] , [46] , [47] , [48] , [49] , [50] . Although detected in the placenta, PRAMEF12 is mostly expressed in adult germ cells and genetic ablation has a sterile phenotype in male, but not female, mice. Whole-mount staining of Pramef12 HA/mCherry transgenic testes indicates that PRAMEF12 is co-expressed with PLZF in most, but not all, undifferentiated spermatogonia. Despite substantial progress in investigating male germline stem cell maintenance, our understanding of the underlying mechanisms that regulate SSC homeostasis remains incomplete. Compared with the reported phenotypes of Id4 , Nanos2, and Plzf knockout mice, the defects in Pramef12 Null mice arise much earlier and are more severe, suggesting critical function(s) for PRAMEF12 in regulating early SSC self-renewal and proliferative expansion. However, the continued presence of PRAMEF12 protein in early differentiating spermatogonia suggests that this germ cell-specific protein also regulates spermatogonial differentiation and meiosis. This is supported by the observation that KIT expression, essential for spermatogonial differentiation and initiation of meiosis [51] , [52] , [53] , is significantly decreased in Pramef12 Null testes. This is associated with decreased numbers of meiotic spermatocytes in P14 and P21 tubules and the failure of the first wave of spermatogenesis to result in mature spermatozoa at P35. The experimental observation that transgenic expression of the recombinant protein restores spermatogenesis and fertility of Pramef12 Null mice, confirms that PRAMEF12 drives SSC functions and spermatogenesis in the mouse testes. Recent studies have reported that PLZF physically interacts with SALL4, and ChIP-seq analysis of PLZF and SALL4 identifies shared regulatory targets ( Bcl6b , Etv5 , Foxo1 , Lhx1 ) involved in SSC self-renewal and differentiation [47] , [54] . To further elucidate PRAMEF12 function, we performed RNA-seq analysis and found that a series of genes involved in SSC self-renewal ( Eomes , Gfra1 , Sall4 , Plzf ), differentiation ( Dmrtb1 , Stra8 , Kit , Sohlh1 , Sohlh2 ) and spermatogenesis ( Piwil2 , Dazl , Ddx4 ) were significantly downregulated in Pramef12 Null testes. These observations suggest that cytoplasmic PRAMEF12 participates in gene activation and acts upstream of genes involved in SSC self-renewal and differentiation. However, unlike cytoplasmic NANOS2 that binds RNA [55] , PRAMEF12 does not have RNA-binding motifs and it remains unclear how PRAMEF12 regulates gene expression. Based on analysis of ID4-positive spermatogonia and expression of other markers in a subset of A s spermatogonia, a hierarchical model has been proposed that supports heterogeneity among SSCs and undifferentiated spermatogonia [9] , [10] . To profile the transcriptome-wide signatures during germline stem cell development and how PRAMEF12 effects this process, we performed focused re-clustering of Pramef12 Het and Pramef12 Null spermatogonial cells. Based on our scRNA-seq data, we find that: (1) four spermatogonial states (SPG1-4) follow a continuous differentiation trajectory and that Pramef12 deficiency impairs germline stem cell development as evidenced by decreased percentages of differentiated cells in SPG3/4 states; (2) Pramef12 deficiency disrupts SSC maintenance- and differentiation-related genes; and (3) the percentage of spermatogonia expressing SSC maintenance-related genes are markedly reduced in Pramef12 Null cells. A recent study reported the developmental trajectory of SSCs and their prospermatogonial precursors by scRNA-seq analysis [38] . To define the SSC fate in the absence of PRAMEF12, we combined the scRNA-seq data on germ cells from P0, P3, and P6 testes with our scRNA-seq data on P7 Pramef12 Het and Pramef12 Null germ cells and compared the transcriptome signatures. These analyses further validate our observations that Pramef12 deficiency severely impairs stem cell potential and blocks stem cell differentiation. In summary, our investigations introduce PRAMEF12 as a newly identified cytoplasmic factor that is required for spermatogonial maintenance and is essential for spermatogenesis and fertility. Not only do these findings provide new insights into molecular mechanisms that regulate SSC homeostasis and differentiation, they also provide a better understanding of male germline stem cell biology, which may translate into treatment of human male infertility. Animals All animal studies were performed in accordance with guidelines of the Animal Care and Use Committee of the National Institutes of Health under a Division of Intramural Research, NIDDK approved animal study protocol (protocol numbers K018LCDB18 and K044LCDB19). Generation of Pramef12 Null mice by CRISPR/Cas9 The guide RNA sequence (5′-GGCTTTGCATTGCGAGCTGT-3′) was designed to target DNA sequence downstream of the Pramef12 start codon. Double-stranded synthetic DNA was cloned into pDR274 (Addgene, #42250) expressing a single guide RNA (sgRNA). After linearization by digestion with DraI, the DNA fragment was purified with PCR Clean-up Kit (Clontech Laboratories) and transcribed using AmpliScribe T7-Flash Transcription Kit (Lucigen). Cas9 mRNA (Addgene #42251) was generated by linearization with PmeI, purified with PCR clean-up kit, and transcribed with mMESSAGE mMACHINE T7 Kit (Thermo Fisher Scientific). After transcription, the sgRNA and Cas9 mRNA were purified with MEGAclear Transcription Clean-Up Kit (Thermo Fisher Scientific). Hormonally stimulated B6D2 F1 (C57LB/6 × DBA2) female mice were mated to B6D2 F1 male mice and zygotes were collected from oviducts at embryonic day 0.5 (E0.5). sgRNA (50 ng μl − 1 ) and Cas9 mRNA (100 ng μl − 1 ) were mixed and injected into the zygotes in M2 medium. Injected zygotes were cultured in KSOM (37 °C, 5% CO 2 ) to the two-cell embryo stage. Two-cell embryos were transferred into the oviducts of pseudo-pregnant ICR female mice at E0.5. 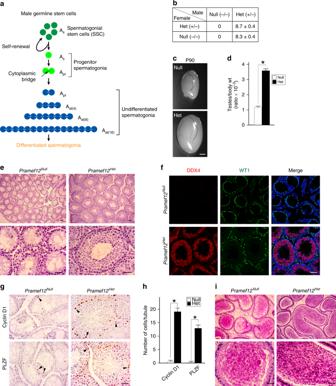Fig. 1 Pramef12is essential for spermatogenesis and male fertility.aThe hierarchy of different cell types of spermatogonia during SSC self-renewal and differentiation. The Asspermatogonia are heterogeneous with SSCs and Asprogenitors. The Asand Aprprogenitors have the potential to become SSCs. Asspermatogonia produce chains of AprAal(4), Aal(8), and Aal(16)undifferentiated spermatogonia that are connected by cytoplasmic bridges and are precursors of differentiated spermatogonia.bFertility of > 3 pairs ofPramef12NullandPramef12Hetmale and female mice mated 1:1. Mean litter sizes ± s.d. are shown with indicated genotypes.cTestes of P90 adultPramef12NullandPramef12Hetmice. Scale bar, 1 mm.dRatios of testis to body weight ofPramef12NullandPramef12Hetmice shown inc. Mean ± s.d,n= 6 biologically independent testes from six different animals. *P=1.44E-08 by two-tailed Student’sttest.eAdult testis sections fromPramef12NullandPramef12Hetmice stained with periodic acid-Schiff (PAS) and hematoxylin.Pramef12Nulltestes are agametic with a Sertoli cell-only phenotype. Scale bar, 50 μm.fImmunofluorescence of P90 adult testes fromPramef12NullandPramef12Hetmice after co-staining with antibodies to DDX4 (germ cells) and WT1 (Sertoli cells) as well as Hoechst 33342 (DNA). Scale bar, 50 μm.gImmunohistochemistry of P90 adult testes fromPramef12NullandPramef12Hetmice after staining with antibodies to cyclin D1 and PLZF. Arrowheads indicate positive-staining spermatogonia. Scale bar, 50 μm.hQuantification of cyclin D1-positive and PLZF-positive spermatogonia inPramef12NullandPramef12Hettestes. Mean ± s.d,n= 3 biologically independent testes from three different animals. *P=1.44E-28 (cyclin D1) and *P=3.19E-26 (PLZF) by two-tailed Student’sttest.iSame ase, but of cauda epididymides. Representative ofn= 6c,n= 3e,f,g,iindependent biological replicates with similar results per condition Primers for genotyping the Pramef12 Null mice are listed in Supplementary Table 1 . Uncropped gels are presented in Supplementary Fig. 8 . Generation of transgenic mice To establish Pramef12 HA/mCherry and Pramef12 FLAG/6xHis/HA transgenic mice, Pramef12 cDNA with N-terminus HA and C-terminus mCherry or with N-terminus FLAG-6xHis and C-terminus HA were inserted into a pmCherry-N1 vector (Clontech). A 3.2 kb DNA sequence upstream of the transcription start site of Pramef12 was amplified from mouse genomic DNA and used as a promoter. A DNA fragment including the promoter and the coding sequence was obtained by digestion of the plasmid with NgoMIV. The transgene was microinjected into the male pronucleus of zygotes and embryo transfers were performed as described above. Genotyping primers for Pramef12 HA/mCherry and Pramef12 FLAG/6xHis/HA transgenic mice were designed to bridge the protein-coding and mCherry sequence or the promoter and protein-coding sequence, respectively (Supplementary Table 1 ). Fertility assay To assess fertility, pairs of Pramef12 Null and Pramef12 Het female mice were co-caged with either a control Pramef12 Het or homozygous Pramef12 Null male mouse for 6 months. The average number of pups per litter was quantified and at least three mating cages were set up for each genotype. A similar approach was used to assess the fertility of Pramef12 Null and Pramef12 Het rescued by the presence of a transgene expressing recombinant PRAMEF12. RNA isolation and quantitative real-time RT-PCR Total RNA was isolated from mouse tissues using RNeasy Mini Kit (Qiagen) and cDNA was synthesized with SuperScript III First-Strand Synthesis System (Thermo Fisher Scientific). Quantitative RT-PCR was performed using iTaq Universal SYBR Green Supermix (Bio-Rad) and QuantStudio 6 Flex Real-Time PCR System (Thermo Fisher Scientific). 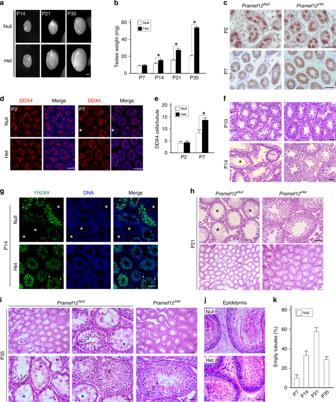Fig. 2 Pramef12is required for the first wave of spermatogenesis.aMorphology of testes from P14, P21, and P35Pramef12NullandPramef12Hetmice. Scale bar, 1 mm.bComparison of testes weight of P7, P14, P21, and P35Pramef12NullandPramef12Hetmice. Mean ± s.d,n= 5 biologically independent testes from five different animals. *P=3.81E-03 (P14), *P=2.38E-06 (P21) and *P=4.84E-08 (P35) by two-tailed Student’sttest. Immunohistochemistrycand immunofluorescencedstaining of DDX4 in the testicular sections from P2 and P7Pramef12NullandPramef12Hetmice. The merge indis with Hoechst 33342 stained DNA. Scale bar, 50 μm.eQuantification of DDX4-positive cells per tubules inPramef12NullandPramef12Hettestes at P2 and P7. Mean ± s.d,n= 3 biologically independent testes from three different animals. *P=2.71E-07 by two-tailed Student’sttest.fTesticular sections of P10 and P14Pramef12NullandPramef12Hetmice were stained with periodic acid-Schiff (PAS) and hematoxylin. Scale bar, 50 μm.gImmunofluorescence staining of γH2AX in testicular sections from P14Pramef12NullandPramef12Hetmice. DNA was stained with Hoechst 33342. Arrows, pachytene spermatocytes (XY body); asterisks, Sertoli cell-only tubules. Scale bar, 50 μm.h,iPAS staining of P21 and P35 testes inPramef12NullandPramef12Hetmice. The reduction in germ cell number becomes notable with the appearance of more agametic tubules (asterisks). Spermatogonia, 1; spermatocytes, 2; spermatids, 3; and elongated spermatozoa, 4; asterisks, agametic tubules. Scale bar, 50 μm.jSame asi, but of cauda epididymides.kPercentage of agametic tubules inPramef12Nulltestes from P7 to P35.Pramef12Hetcontrol testes contain no empty tubules. Mean ± s.d,n= 3 biologically independent testes from 3 different animals at each age point. Representative ofn= 5a,n= 3c,d,f–jindependent biological replicates with similar results per condition The primers used in these experiments are listed in Supplementary Table 2 . The relative abundance of each transcript was calculated by the 2 −ΔΔ Ct normalized to endogenous β-actin expression [56] . Uncropped gels of Fig. 4a are presented in Supplementary Fig. 8 . Histology and IF Mouse testes and epididymides were fixed in Bouin’s solution or 4% paraformaldehyde (PFA) overnight at 4 °C for histology or immunostaining, respectively. Samples were embedded in paraffin, sectioned (5 μm-thick) and mounted on slides prior to staining with periodic acid-Schiff (PAS) and hematoxylin. Cell apoptosis was measured by terminal deoxynucleotidyl transferase-mediated deoxyuridine triphosphate (TUNEL) assay using an In situ Apoptosis Detection Kit (Millipore) according to the manufacturer’s instructions. 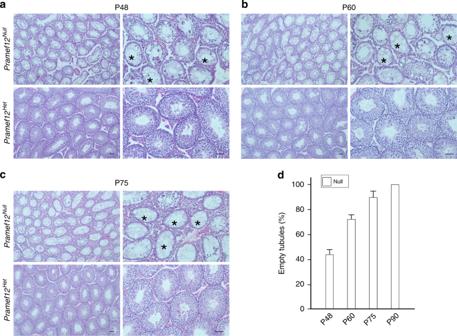Fig. 3 Further evaluation of spermatogenic phenotype ofPramef12Nullmice.aTesticular sections of P48Pramef12NullandPramef12Hetmice were stained with periodic acid-Schiff (PAS) and hematoxylin. Asterisks, agametic tubules. Scale bar, 50 μm.bSame asa, but of P60 testes.cSame asa, but of P75 testes.dStatistical analysis of empty tubules from P48 to P90Pramef12Nullmice. Mean ± s.d,n= 3 biologically independent testes from three different animals at each age point. Representative ofn= 3a–cindependent biological replicates with similar results per condition After de-waxing, rehydration, and antigen retrieval with 0.01% sodium citrate buffer (pH 6.0) (Sigma Aldrich), tissue sections were blocked with SuperBlock Blocking Buffer containing 0.05% Tween-20 at RT for 1 h and incubated with primary antibodies (Supplementary Table 3 ) overnight at 4 °C. For IF, secondary antibodies conjugated to Alexa Fluors (Supplementary Table 3 ) were used to detect the antigen and DNA was stained with Hoechst 33342. For immunohistochemistry, ImmPRESS Polymer Detection Kit (Vector Laboratories) and diaminobenzidine were used to detect antibody binding. For whole-mount staining, freshly isolated testes were fixed in 4% PFA overnight at 4 °C, permeabilized in SuperBlock Blocking Buffer containing 5% donkey serum, 3% bovine serum albumin, 0.5% Triton X-100 and 0.05% Tween-20 overnight at 4 °C and then incubated with primary antibodies (Supplementary Table 3 ) for 3–5 days at 4 °C. Secondary antibodies conjugated to Alexa Fluors (Supplementary Table 3 ) were incubated with the testes for an additional 3–5 days at 4 °C. After washing in PBS, testes were mounted with PBS on the slides. Bright field images were obtained with an inverted microscope (AxioPlan 2; Carl Zeiss) and fluorescent images were captured with a confocal microscope (LSM 780; Carl Zeiss). Immunoblot Total protein was extracted in 1 × LDS sample buffer with 1 × NuPAGE Sample Reducing Agent (Thermo Fisher Scientific). Proteins were separated on 4–12% Bis-Tris gels and electrophoretically transferred to polyvinylidene difluoride membranes. The membranes were blocked with 5% nonfat milk in Tris-buffered saline containing 0.05% Tween-20 (TBST) at RT for 1 h and probed with primary antibodies (Supplementary Table 3 ) overnight at 4 °C. The membranes then were washed three times with TBST and incubated (1 h, RT) with secondary antibodies (Supplementary Table 3 ), washed with TBST and developed using SuperSignal West Dura Extended Duration Substrate (Thermo Fisher Scientific). Signals were detected with PXi Touch (SYNGENE) or Hyperfilm ECL (GE Healthcare) according to the manufacturer’s instructions. Uncropped blots are presented in Supplementary Fig. 8 . Isolation of single testicular cells by FACS Single cells were isolated according to published protocols [57] , [58] with minor modifications. In brief, P7 Pramef12 Null and Pramef12 Het testes were collected and de-capsulated in Hank’s Balanced Salt Solution (HBSS, Gibco). Testicular tubules were digested in 15 ml conical tubes containing 5 ml (1 mg ml − 1 ) of collagenase (Type IV, Sigma Aldrich)/DNase I (Sigma Aldrich) solution in HBSS at 37 °C with gentle agitation for 15 min. The dispersed tubules were then digested with 0.25% trypsin/EDTA and DNase I at 37 °C with gentle agitation for 7 min. When most of the cells were dispersed, trypsin was neutralized by adding 20% fetal bovine serum (FBS). The cell suspensions were filtered through a pre-wetted 70-μm cell strainer (Corning) and were pelleted by centrifugation at 300 × g for 5 min. The cell pellets were resuspended in HBSS with 15% FBS at a concentration of 1 × 10 6 cells ml − 1 . For FACS analysis, the cells were stained with 1 μg ml − 1 DAPI to exclude dead cells and stained with DRAQ5 dye (Thermo Fisher Scientific) to quantify DNA content, filtered through a 40-μm cell strainer (Corning) before loading on a MoFlo Astrios EQ high speed cell sorter (Beckman Coulter). Flow data analysis was performed using Summit software V6.3.016900 (Beckman Coulter). Sorting strategies for isolation vital single testicular cells were shown in Supplementary Fig. 9 . Cells were sorted into HBSS supplemented with 15% FBS and freshly isolated cells were immediately used for scRNA-seq library preparation. FACS experiments were performed at NINDS Flow Cytometry Core Facility in a BSL2 enclosure. RNA-seq library preparation Total RNA was isolated using RNeasy Mini Kit and mRNA was purified by Dynabeads mRNA Purification Kit (Thermo Fisher Scientific). First-strand cDNA was synthesized with SuperScript III Reverse Transcriptase and the second strand was synthesized in 100 μl containing: 20 μl of the first-strand cDNA synthesis mix, 10 μl of 10 × second strand buffer (500 m m Tris-HCl, pH 7.5; 50 m m MgCl 2 ; 10 m m DTT), 3 μl of dNTP mix (10 m m ), 1 μl of RNaseH (2 U μl − 1 ), 5 μl of DNA Pol I (10 U μl − 1 ) and 61 μl H 2 O. The mixture was incubated for 2 h at 16 °C. The libraries were constructed with Nextera DNA Sample Preparation Kit (Illumina) per the manufacturer’s protocol in which double-strand cDNA was fragmented, subjected to adapter ligation and amplified. The final PCR amplified libraries were sequenced at the NIDDK Genomic Core Facility. scRNA-seq library preparation scRNA-seq libraries were prepared using single-cell 3′ reagent kits v2 (10× Genomics) according to the manufacturer’s instructions at the NHLBI Core Facility. In brief, cells obtained from FACS were mixed with a suspension containing barcoded beads and UMI (unique molecular identifier) elements that allow specific tagging of messenger RNA. After partitioning thousands of cells into nanoliter-scale Gel Bead-In-EMulsions (GEMs) and barcoding, full-length barcoded cDNA is then amplified by PCR to generate sufficient mass for library construction. Libraries were constructed by fragmentation, end repair, A-tailing, adaptor ligation, and index PCR. After ensuring adequate quality of the cDNA libraries, the samples were sequenced at the NHLBI Genomic Core Facility. RNA-seq analysis Raw sequence reads were trimmed with cutadapt v1.16 to remove any adapters while performing light quality trimming using parameters -q 20 -a AGATCGGAAGAGC–minimum-length 25. Trimmed reads were mapped to the mm10 reference genome using HISAT v2.1.0 with default parameters [59] and multimapping reads were filtered using SAMtools v1.7 [60] . Uniquely aligned reads were then mapped to gene features using subread featureCounts v1.6.1 with default parameters [61] . Differential expression between groups of samples was tested in R v3.4.1 with DESeq2 v1.18.1 [62] . scRNA-seq data processing Raw read processing was carried out using the CellRanger Single-Cell Software Suite (version 3.0.0, 10× Genomics Inc., CA). In brief, the demultiplexed FASTQ files (26 bp Cell barcode and UMI Read1, 8 bp i7 index, and 100 bp Read2) were generated using the CellRanger mkfastq command. The primary data analyses that included alignment, filtering, barcode counting and UMI quantification for determining gene transcript counts per cell (generated a gene-barcode matrix), quality control, clustering and statistical analysis were performed using CellRanger count command. Gene positions were annotated using Ensembl build 93 and filtered for biotype (only protein-coding, long intergenic non-coding RNA, antisense, immunoglobulin or T-cell receptor). Single-cell transcriptomes to identify cell types Raw gene expression matrices generated per sample using CellRanger (version 3.0.0) were imported into R (version 3.5.0) and converted to a Seurat object using the Seurat R package (version 2.3.4) [63] . Cells that had either fewer than 300 expressed genes, over 30,000 or below 1619 UMIs, or over 15% UMIs derived from mitochondrial genome were discarded. For the remaining 10,060 cells, gene expression matrices were normalized to total cellular read count and to mitochondrial read count using negative binomial regression method implemented in Seurat RegressOut function. Cell Cycle scores were also calculated using Seurat CellCycleScoring function since the Cell cycle phase effect was observed. The gene expression matrices were then further normalized to cell cycle scores. The variably expressed genes were selected from the normalized data. The gene that had a normalized expression value between 0.13 and 8, a quantile-normalized variance exceeding 0.9, and was not a mitochondrial or ribosome protein-coding genes was defined as highly variably genes (HVG). 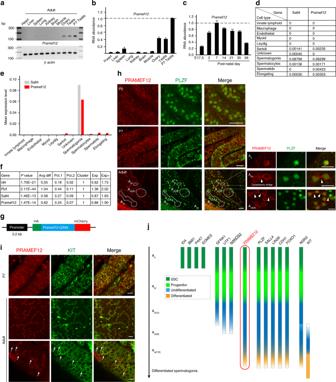Fig. 4 PRAMEF12 is specifically expressed in spermatogonia.a–cAbundance ofPramef12transcripts in different adult tissues and P7 testesa,band E17.5-P56 testescwas determined by RT-PCRaor qRT-PCRb,cusingβ-actinas a control. Molecular mass, left ina. The highest expression level ofPramef12relative toβ-actinwas set to 1 inb,c. Mean ± s.d,n= 3 biologically independent samples per condition.d–fAnalyses of the abundance ofPramef12transcripts in 11 testicular cell typesd,eand in cluster 1 of re-clustered germ cellsfbased on previously reported scRNA-seq data in adult mouse testes34. Numbers indand theYaxis inereflect the averaged UMIs detected in each individual cell. After re-clustering germ cells,Id4,Plzf,andSall4serve as positive controls and, likeSall4,Pramef12was primarily enriched in the spermatogonial cluster 1, which corresponds to undifferentiated spermatogoniaf.Pvalue infwas obtained from the published scRNA-seq data34. Avg diff, log2-scale fold change. Percent of cells expressing gene in cluster 1 (Pct.1) or in non-cluster 1 cells (Pct.2). Exp and Exp + reflect mean expression of the marker in all cells of this cluster and in the marker-positive cells of this cluster, respectively.gSchematic representation of transgene expressingHAPramef12mCherrycDNA driven by thePramef12promoter (3.2 kb).hWhole-mount staining of P2, P7 and adultPramef12HA/mCherrytestes with antibodies to mCherry (left), PLZF (middle) and merged (right). Scale bar, 50 μm. Examples of As, Apr, and Aalundifferentiated spermatogonia in adult testes (dotted circles) and enlarged (right panels). Arrowheads, high-light cytoplasmic location. Scale bar, 20 μm.iSame ashfor P7 and adult testes, but with antibodies to mCherry (left), KIT (middle) and merged (right). Arrows, high-light co-localization of the two markers.jThe expression profile of intracellular molecular markers for male germline cells. Except for NANOS2 (underlined), PRAMEF12 (underlined, red) is unique in its cell type specificity and is largely enriched in undifferentiated spermatogonia. Representative ofn= 3a,h,iindependent biological replicates with similar results per condition The resulting 1334 HVGs were used as features for dimensionality reduction and clustering. The Seurat RunPCA and JackStraw functions was performed to select principal components (PCs), which hold the most differences to separate the cells. The RunTSNE function with default setting was then applied to plot the selected significant PCs. We further performed the batch effect correction using Hormany [64] because a batch effect between two samples was observed. The RunTSNE function with default setting was applied to plot the first 25 Harmony aligned coordinates. The FindClusters function with resolution = 0.4 parameter was carried out to cluster cells into different groups. The canonical marker genes were applied to annotated cell clusters to known biological cell types. Re-clustering of the germ cell types To identify sub-clusters within spermatogonia-specific cell type, we re-analyzed cells that belonged to spermatogonial cell type separately. Specifically, we selected the HVGs for spermatogonial cell type as described above, and then applied principle component analysis on the selected HVGs for dimensionality reduction. To identify which principle components were informative, we determined statistical significance of PCA scores using Seurat function JackStraw , selecting those principle components with P value < 0.5. 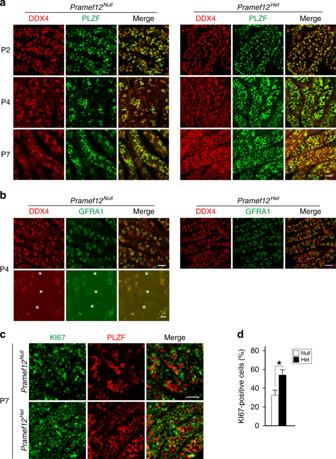Fig. 5 Essential role of PRAMEF12 in early spermatogenic maintenance.aImmunofluorescence of whole-mount testes from P2, P4, and P7Pramef12Null(left group) andPramef12Het(right group) mice after staining with antibodies to DDX4 (left) or PLZF (middle) and merged (right). The number of PLZF-positive spermatogonia was comparable in P2Pramef12NullandPramef12Hettubules and significantly decreased inPramef12Nulltubules as early as at P4, although still present at P7. Scale bar, 50 μm.bSame asa, but with antibodies to GFRA1 (co-receptor for GDNF) at P4. Asterisks, agametic tubules.cSame asa, but with antibodies to KI67 (marker of mitosis) and PLZF using whole-mount testes fromPramef12Null(top) andPramef12Het(bottom) mice at P7.dThe percent of KI67+; PLZF+double-positive among the total PLZF+single-positive spermatogonia in P7Pramef12NullandPramef12Hettubules. At least six random regions of individual testis were counted from at least three different mice. Mean ± s.d,n= 3 biologically independent samples per condition. *P=5.89E-23 by two-tailed Student’sttest. Representative ofn= 3a–cindependent biological replicates with similar results per condition The batch effect correction was also performed as described above. First 20 Harmony aligned coordinates further summarized to UMAP dimensionality reduction using the default of the UMAP function RunUMAP [37] . Using the graph-based clustering approach implemented in the FindClusters function of the Seurat package, with a conservative resolution of 0.8 and otherwise default parameters, cells were re-clustered by UMAP aligned coordinates. Identification of marker genes To identify marker genes for these nine cell types, we compared the gene expression values of cells from the cluster of interest with that of cells from the rest of clusters using the Seurat FindMarkers function with default parameter of Wilcoxon rank-sum test. Marker genes were defined based on the following criteria: (1) the average expression value in the cluster of interest was at least 2.5-fold higher than the average expression in the rest of clusters; (2) there are > 10% of cells in the cluster of interest that were detectable; and (3) marker genes should have the highest mean expression in the cluster of interest compared with the rest of clusters. Statistical analysis Unless otherwise noted, data are presented as the mean ± s.d. 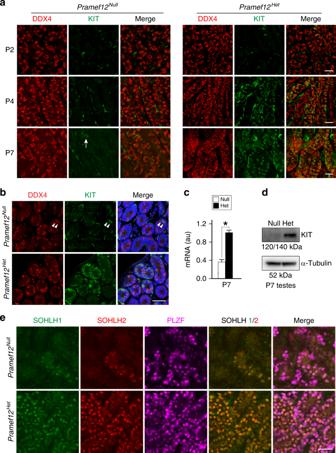Fig. 6 Essential role of PRAMEF12 in spermatogonial differentiation.aImmunofluorescence of whole-mount testes from P2, P4, and P7Pramef12NullandPramef12Hetmice after staining with antibodies to DDX4 (left) or KIT (middle) and merged (right). KIT-positive spermatogonia were rarely detected at P2 in eitherPramef12NullorPramef12Hettubules but were present at P4 and increased at P7 inPramef12Hettubules. Few KIT-positive spermatogonia (arrow) were observed in P7Pramef12Nulltubules. Scale bar, 50 μm.bImmunohistochemistry of sections from P7Pramef12Null(top panels) andPramef12Het(bottom panels) testes after staining with antibodies to DDX4 (left) or KIT (middle) and merged with Hoechst 33342 to stain DNA (right). Arrowheads, KIT-positive cells inPramef12Nulltestes. Scale bar, 50 μm.cQuantitative real-time RT-PCR ofKitmRNA abundance in P7Pramef12NullandPramef12Hettestes usingβ-actinas an internal load control and setting the abundance inPramef12Hettestis to 1. Mean ± s.d,n= 3 biologically independent samples per condition. *P=1.43E-05 by two-tailed Student’sttest.dImmunoblot of KIT protein in P7Pramef12NullandPramef12Hettestes using α-tubulin as a load control.eSame asa, but with antibodies to SOHLH1, SOHLH2, and PLZF. The number of spermatogonia positive for SOHLH1 and SOHLH2 was significantly reduced in P7Pramef12Nulltubules (top panels). Representative ofn= 3a,b,d,eindependent biological replicates with similar results per condition The two-tailed Student’s t test was used to calculate Ρ values. Ρ < 0.05 was considered statistically significant. 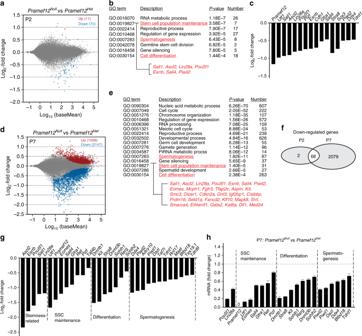Fig. 7 Pramef12deficiency alters expression patterns of spermatogenic genes.aMA plot (log ratio RNA abundance versus abundance) of RNA-seq data fromPramef12NullandPramef12Hettestes at P2. 11 genes and 70 genes were upregulated and downregulated, respectively, inPramef12Nulltestes using adjustedP<0.1 as the cut off.bGene ontology of downregulated genes in P2Pramef12Nulltestes. Genes that support stem cell population maintenance indicated in red text fly-out. GO terms were obtained by GOrilla analysis.Pvalue was obtained from the data by GOrilla analysis.cGenes related to stem cell maintenance and differentiation that were significantly downregulated (log2-fold change) in P2Pramef12Nulltestes.dSame asa, but at P7. In all, 1599 genes and 2147 genes were upregulated and downregulated inPramef12Nulltestes, respectively.eSame asb, but at P7.Pvalue was obtained from the data by GOrilla analysis.fVenn diagram depicting the overlap of downregulated genes determined at two developmental time points, P2 and P7.gRNA-seq results of selected transcripts (log2-fold change) related to SSC maintenance, differentiation and spermatogenesis that were significantly downregulated in P7Pramef12Nulltestes.hQuantitative RT-PCR validation of downregulated genes involved in SSC maintenance, differentiation and spermatogenesis inPramef12Nulltestes at P7. For comparison, the abundance (relative toβ-actin) of each gene inPramef12Hetcontrol mice was set to 1. Data are presented as mean ± s.d forn= 3 biologically independent samples per condition 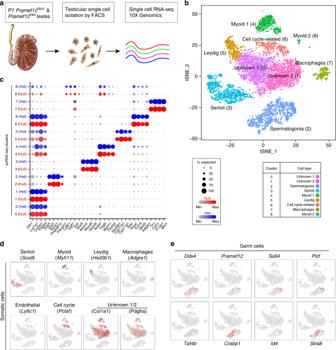Fig. 8 Single-cell transcriptome ofPramef12HetandPramef12Nulltesticular cells.aSchematic illustration of the workflow for scRNA-seq analysis.btSNE and clustering analysis of combined single-cell transcriptome data from P7Pramef12HetandPramef12Nulltesticular cells. Each dot represents a single-cell and cell clusters are distinguished by colors.cDotplot for expression of selected marker genes across all identified cell types.dGene expression patterns of selected somatic cell marker genes projected on the tSNE plots.eExpression patterns of marker genes for germ cells visualized in tSNE plots.Pramef12is exclusively expressed in germ cell population but not in somatic cell populations 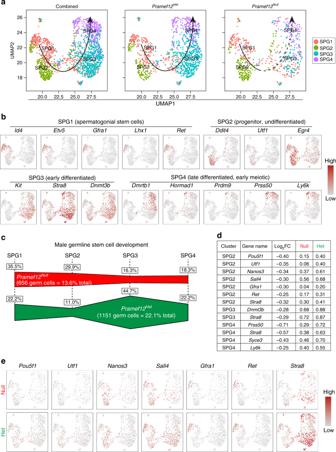Fig. 9 Transcriptome-wide signatures of germline stem cell development.aFocused analysis (UMAP clustering and pseudotime ordering) of combined (left),Pramef12Het(middle), andPramef12Null(right) germ cells documented four biological subtypes following the order of SPG1 to SPG4 (state 1 to state 4).bGene expression patterns of selected marker genes corresponding to each cellular state on the UMAP plots.cSummary schematic depicting the percentage of spermatogonia in each cellular state inPramef12NullandPramef12Hettestes.Pramef12deficiency significantly impairs germline stem cell development as determined by the decreased percentage of differentiated cells in SPG3 and SPG4.dDifferentially expressed genes (DEGs) betweenPramef12NullandPramef12Hetcells in SPG2, SPG3, and SPG4. Log2FC, log2-fold change. Null and Het indicate the percentage of cells in which the gene was detected inPramef12NullandPramef12Hetsamples, respectively.eUMAP plots of the expression patterns of selected DEGs in SPG2 subtype inPramef12NullandPramef12Hetsamples 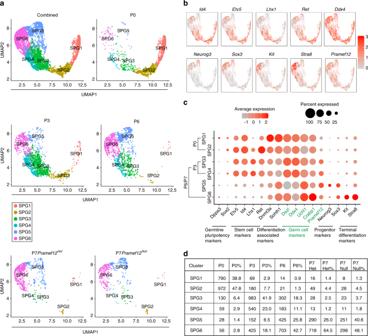Fig. 10 Spermatogonial stem cell fates inPramef12Nullmale mice.aUMAP clustering of the combined germ cells including P0, P3, P6, P7Pramef12Het, andPramef12Nullsamples documented six biological subtypes following a developmental trajectory of SPG1 to SPG6 (upper left). Five additional UMAP plots specific to each individual sample (right and below).bGene expression patterns of selected spermatogonial marker genes corresponding to each cellular state on the UMAP plots: SPG1 (Id4,Etv5,Ret); SPG2 (Id4,Etv5,Lhx1,Ret); SPG3 (Id4,Etv5,Lhx1,Ret); SPG4 (Id4,Etv5,Lhx1,Ret); SPG5 (Neurog3,Sox3); and SPG6 (Kit,Stra8).cDotplot representation of average scaled expression and the percentage of cells within each cluster for selected marker genes across all ages and cell types.dTable of the distribution and the percentage of the cells within each cluster and each sample Reporting summary Further information on research design is available in the Nature Research Reporting Summary linked to this article.